Doping dependence of spin excitations and its correlations with high-temperature superconductivity in iron pnictides High-temperature superconductivity in iron pnictides occurs when electrons and holes are doped into their antiferromagnetic parent compounds. Since spin excitations may be responsible for electron pairing and superconductivity, it is important to determine their electron/hole-doping evolution and connection with superconductivity. Here we use inelastic neutron scattering to show that while electron doping to the antiferromagnetic BaFe 2 As 2 parent compound modifies the low-energy spin excitations and their correlation with superconductivity (<50 meV) without affecting the high-energy spin excitations (>100 meV), hole-doping suppresses the high-energy spin excitations and shifts the magnetic spectral weight to low-energies. In addition, our absolute spin susceptibility measurements for the optimally hole-doped iron pnictide reveal that the change in magnetic exchange energy below and above T c can account for the superconducting condensation energy. These results suggest that high- T c superconductivity in iron pnictides is associated with both the presence of high-energy spin excitations and a coupling between low-energy spin excitations and itinerant electrons. In conventional Bardeen-Cooper-Schrieffer (BCS) superconductors [1] , superconductivity occurs when electrons form coherent Cooper pairs below the superconducting transition temperature T c . Although the kinetic energy of paired electrons increases in the superconducting state relative to the normal state, the reduction in the ion lattice energy is sufficient to give the superconducting condensation energy ( E c =− N (0)Δ 2 /2 and Δ≈2 ħ ω D , where N (0) is the electron density of states at zero temperature, ħ ω D is the Debye energy, and V 0 is the strength electron-lattice coupling) [1] , [2] , [3] . For iron pnictide superconductors derived from electron or hole-doping of their antiferromagnetic (AF) parent compounds [4] , [5] , [6] , [7] , [8] , [9] , the microscopic origin for superconductivity is unclear. Although spin excitations arising from quasiparticle excitations between the hole pockets near Γ and electron pockets at M in reciprocal space have been suggested as the microscopic origin for superconductivity [10] , [11] , orbital fluctuations may also induce superconductivity in these materials [12] . Here we use inelastic neutron scattering (INS) to systematically map out energy and wave vector dependence of the spin excitations in electron and hole-doped iron pnictides with different superconducting transition temperatures. By comparing the outcome with previous spin wave measurements on the undoped parent compound BaFe 2 As 2 (ref. 13 ), we find that high- T c superconductivity only occurs for iron pnictides with low-energy (≤25 meV or ~6.5 k B T c ) itinerant electron-spin excitation coupling and high-energy (>100 meV) spin excitations. Since our absolute spin susceptibility measurements for optimally hole-doped iron pnictide reveal that the change in magnetic exchange energy below and above T c [14] , [15] can account for the superconducting condensation energy, we suggest that the presence of both high-energy spin excitations giving rise to a large magnetic exchange coupling J and low-energy spin excitations coupled to the itinerant electrons are important for high- T c superconductivity in iron pnictides. For BCS superconductors, the superconducting condensation energy E c and T c are controlled by the strength of the Debye energy ħ ω D and electron-lattice coupling V 0 (refs 1 , 2 , 3 ). A material with large ħ ω D and lattice exchange coupling is a necessary but not a sufficient condition to have high- T c superconductivity. On the other hand, a soft metal with small ħ ω D (such as lead and mercury) will also not exhibit superconductivity with high- T c . For unconventional superconductors such as iron pnictides, the superconducting phase is derived from hole and electron doping from their AF parent compounds [4] , [5] , [6] , [7] , [8] , [9] . Although the static long-range AF order is gradually suppressed when electrons or holes are doped into the iron pnictide parent compound such as BaFe 2 As 2 (refs 5 , 6 , 7 , 8 , 9 ), short-range spin excitations remain throughout the superconducting phase and are coupled directly with the occurrence of superconductivity [16] , [17] , [18] , [19] , [20] , [21] , [22] , [23] , [24] , [25] . For spin excitations-mediated superconductors, the superconducting condensation energy should be accounted for by the change in magnetic exchange energy between the normal (N) and superconducting (S) phases at zero temperature. For an isotropic t - J model [26] , Δ E ex ( T )=2 J [‹ S i + x · S i › N −‹ S i + x · S i › S ], where J is the nearest neighbour magnetic exchange coupling and ‹ S i + x · S i › is the dynamic spin susceptibility in absolute units at temperature T [14] , [15] . Since the dominant magnetic exchange couplings are isotropic nearest neighbour exchanges for copper oxide superconductors [27] , [28] , the magnetic exchange energy Δ E ex ( T ) can be directly estimated using the formula through carefully measuring of J and the dynamic spin susceptibility in absolute units between the normal and superconducting states [29] , [30] , [31] . For heavy Fermion superconductor such as CeCu 2 Si 2 , one has to modify the formula to include both the nearest neighbour and next nearest neighbour magnetic exchange couplings appropriate for the tetragonal unit cell of CeCu 2 Si 2 to determine Δ E ex ( T ) (ref. 32 ). In the case of iron pnictide superconductors [5] , [6] , [7] , [8] , [9] , the effective magnetic exchange couplings in their parent compounds are strongly anisotropic along the nearest neighbour a o and b o axis directions of the orthorhombic structure (see inset in Fig. 1a ) [13] , [33] , [34] . Although the electron doping induced lattice distortions in iron pnictides [35] may affect the effective magnetic exchange couplings [36] , our INS experiments on optimally electron-doped BaFe 1.9 Ni 0.1 As 2 indicate that the high-energy spin excitations, which determines the effective magnetic exchange couplings [13] , [33] , [34] , are weakly electron doping-dependent [24] . 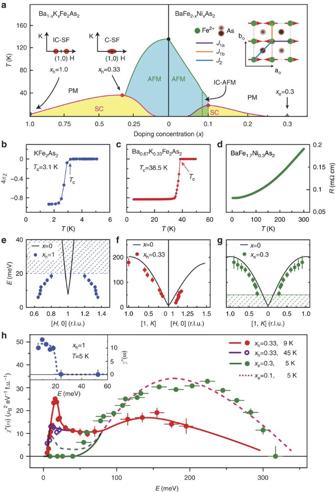Figure 1: Summary of transport and neutron scattering results. (a) The electronic phase diagram of electron and hole-doped BaFe2As2(ref.9). The right inset shows crystal and AF spin structures of BaFe2As2with marked the nearest (J1a,J1b) and next nearest neighbor (J2) magnetic exchange couplings. The left insets show the evolution of low-energy spin excitations in Ba1−xKxFe2As2. (b,c) Temperature dependence of magnetic susceptibility for our KFe2As2and Ba0.67K0.33Fe2As2. (d) Temperature dependence of the resistivity for BaFe1.7Ni0.3As2. (e–g) The filled circles are spin excitation dispersions of KFe2As2at 5 K, Ba0.67K0.33Fe2As2at 9 K, and BaFe1.7Ni0.3As2at 5 K, respectively. The shaded areas indicate vanishing spin excitations and the solid lines show spin wave dispersions of BaFe2As2(ref.13). (h) Energy dependence of χ″(ω) for BaFe1.9Ni0.1As2(dashed line), BaFe1.7Ni0.3As2(green solid circles), Ba0.67K0.33Fe2As2below (solid red circles and solid red line) and above (open purple circles and solid lines)Tc. The inset shows Energy dependence of χ″(ω) for KFe2As2. The vertical error bars indicate the statistical errors of one standard deviation. The horizontal error bars in (h) indicate the energy integration range. Therefore, we can rewrite the relation between the magnetic exchange coupling and the magnetic exchange energy as [15] Figure 1: Summary of transport and neutron scattering results. ( a ) The electronic phase diagram of electron and hole-doped BaFe 2 As 2 (ref. 9 ). The right inset shows crystal and AF spin structures of BaFe 2 As 2 with marked the nearest ( J 1a , J 1b ) and next nearest neighbor ( J 2 ) magnetic exchange couplings. The left insets show the evolution of low-energy spin excitations in Ba 1− x K x Fe 2 As 2 . ( b , c ) Temperature dependence of magnetic susceptibility for our KFe 2 As 2 and Ba 0.67 K 0.33 Fe 2 As 2 . ( d ) Temperature dependence of the resistivity for BaFe 1.7 Ni 0.3 As 2 . ( e – g ) The filled circles are spin excitation dispersions of KFe 2 As 2 at 5 K, Ba 0.67 K 0.33 Fe 2 As 2 at 9 K, and BaFe 1.7 Ni 0.3 As 2 at 5 K, respectively. The shaded areas indicate vanishing spin excitations and the solid lines show spin wave dispersions of BaFe 2 As 2 (ref. 13 ). ( h ) Energy dependence of χ ″ (ω) for BaFe 1.9 Ni 0.1 As 2 (dashed line), BaFe 1.7 Ni 0.3 As 2 (green solid circles), Ba 0.67 K 0.33 Fe 2 As 2 below (solid red circles and solid red line) and above (open purple circles and solid lines) T c . The inset shows Energy dependence of χ ″ (ω) for KFe 2 As 2 . The vertical error bars indicate the statistical errors of one standard deviation. The horizontal error bars in ( h ) indicate the energy integration range. Full size image Here the scattering function S ( Q , E = ħ ω) is related to the imaginary part of the dynamic susceptibility χ ″ ( Q ,ω) via S ( Q ,ω)=[1+ n (ω, T )]χ ″ ( Q ,ω), where [1+ n (ω, T )] is the Bose population factor, Q the wave vector, and E = ħ ω the excitation energy. J 1a is the effective magnetic coupling strength between two nearest sites along the a o direction, while J 1b is that along the b o direction and J 2 is the coupling between the next nearest neighbour sites (see inset in Fig. 1a ) [13] . To determine how high- T c superconductivity in iron pnictides is associated with spin excitations, we consider the phase diagram of electron and hole-doped iron pnictide BaFe 2 As 2 ( Fig. 1a ) [9] . In the undoped state, BaFe 2 As 2 forms a metallic low-temperature orthorhombic phase with collinear AF structure as shown in the inset of Fig. 1a . INS measurements have mapped out spin waves throughout the Brillouin zone and determined the effective magnetic exchange couplings [13] . Upon doping electrons to BaFe 2 As 2 by partially replacing Fe with Ni to induce superconductivity in BaFe 2− x Ni x As 2 with maximum T c ≈20 K at x e =0.1 (ref. 37 ), the low-energy (<80 meV) spin waves in the parent compounds are broadened and form a neutron spin resonance coupled to superconductivity [20] , [21] , [22] , [23] , while high-energy spin excitations are weakly affected [24] . With further electron doping to x e ≥0.25, superconductivity is suppressed and the system becomes a paramagnetic metal ( Fig. 1a ) [37] . For hole-doped Ba 1− x K x Fe 2 As 2 (ref. 38 ), superconductivity with maximum T c =38.5 K appears at x h ≈0.33 (ref. 5 ) and pure KFe 2 As 2 at x h =1 is a T c =3.1 K superconductor [6] . In order to determine how spin excitations throughout the Brillouin zone are correlated with superconductivity in iron pnictides, we study optimally hole-doped Ba 0.67 K 0.33 Fe 2 As 2 ( T c =38.5 K, Fig. 1c ), pure KFe 2 As 2 ( T c =3 K, Fig. 1b ), and nonsuperconducting electron-overdoped BaFe 1.7 Ni 0.3 As 2 ( Fig. 1d ). If spin excitations are responsible for mediating electron pairing and superconductivity, the change in magnetic exchange energy between the normal and superconducting state should be large enough to account for the superconducting condensation energy [15] . From density functional theory (DFT) calculations, one finds that Fermi surfaces for the undoped parent compound BaFe 2 As 2 consist of hole-like pockets near the Brillouin zone centre and electron pockets near the zone corner ( Fig. 2a ) [10] . 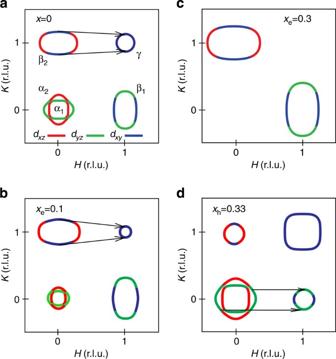Figure 2: Schematics of Fermi surface evolution as a function of Ni-doping for BaFe2−xNixAs2and for Ba0.67K0.33Fe2As2. (a–c) Evolution of Fermi surfaces with Ni-dopings ofxe=0,0.1,0.3. Thedxz,dyz, anddxyorbitals for different Fermi surfaces are coloured as red, green and blue, respectively. (d) Fermi surfaces for Ba0.67K0.33Fe2As2. Figure 2a–d shows the evolution of Fermi surfaces as a function of electron- and hole-doping obtained from the tight-binding model of Graser et al. [39] When electrons are doped into the parent compounds, the hole Fermi surfaces decrease in size while the electron pocket sizes increase ( Fig. 2b ) [40] . As a consequence, quasiparticle excitations between the hole and electron Fermi surfaces form transversely elongated spin excitations that increase with increasing electron doping [23] , [24] , [25] . For electron-overdoped iron pnictides, the hole pockets sunk below the Fermi surface ( Fig. 2c ) [40] . The absence of interband transition between the hole and electron Fermi surfaces is expected to result in a complete suppression of the low-energy spin excitations at the AF ordering wave vector. This is indeed confirmed by nuclear magnetic resonance experiments on electron overdoped Ba(Fe 1− x Co x ) 2 As 2 (ref. 41 ). For optimally hole-doped iron pnictide Ba 0.67 K 0.33 Fe 2 As 2 (inset in Fig. 1a ), DFT theory based on sign reversed quasiparticle excitations between hole and electron pockets ( Fig. 2d ) predicts correctly the longitudinally elongated spin excitations from Q AF =(1,0) [23] , [18] . In addition, INS work on powder [16] , [17] and single crystals [18] of hole-doped Ba 1− x K x Fe 2 As 2 reveal that the low-energy spin excitations are dominated by a resonance coupled to superconductivity. For pure KFe 2 As 2 ( x h =1), low-energy (<14 meV) spin excitations become longitudinally incommensurate from Q AF =(1,0) (inset in Fig. 1a ) [19] . These results, as well as the work on electron-doped iron pnictides [23] , [24] , [25] , have shown that the low-energy spin excitations in iron-based superconductors can be accounted for by itinerant electrons on the hole and electron-nested Fermi surfaces [9] . Figure 2: Schematics of Fermi surface evolution as a function of Ni-doping for BaFe 2− x Ni x As 2 and for Ba 0.67 K 0.33 Fe 2 As 2 . ( a – c ) Evolution of Fermi surfaces with Ni-dopings of x e =0,0.1,0.3. The d xz , d yz , and d xy orbitals for different Fermi surfaces are coloured as red, green and blue, respectively. ( d ) Fermi surfaces for Ba 0.67 K 0.33 Fe 2 As 2 . Full size image Here we use INS to show that the effect of hole-doping to BaFe 2 As 2 is to suppress high-energy spin excitations and transfer the spectral weight to low-energies that couple to the appearance of superconductivity ( Fig. 1h ). The overall spin excitations spectrum in optimally hole-doped superconducting Ba 0.67 K 0.33 Fe 2 As 2 is qualitatively consistent with theoretical methods based on DFT and dynamic mean filed theory (DMFT) [42] . By using the INS measured magnetic exchange couplings and spin susceptibility in absolute units, we calculate the superconductivity-induced lowering of magnetic exchange energy and find it to be about seven times larger than the superconducting condensation energy determined from specific heat measurements for Ba 0.67 K 0.33 Fe 2 As 2 (ref. 43 ). These results are consistent with spin excitations-mediated electron pairing mechanism [15] . For the nonsuperconducting electron-overdoped BaFe 1.7 Ni 0.3 As 2 , we find that while the effective magnetic exchange couplings are similar to that of optimally electron-doped BaFe 1.9 Ni 0.1 As 2 ( Fig. 1g ) [24] , the low-energy spin excitations (<50 meV) associated with the hole and electron pocket Fermi surface nesting disappear ( Fig. 2c ), thus revealing the importance of Fermi surface nesting and itinerant electron-spin excitation coupling to the occurrence of superconductivity ( Fig. 1h ). Finally, for heavily hole-doped KFe 2 As 2 with low- T c superconductivity ( Fig. 1b ), there are only incommensurate spin excitations below ~25 meV possibly due to the mismatched electron-hole Fermi surfaces [19] , [44] and the correlated high-energy spin excitations prevalent in electron-doped and optimally hole-doped iron pnictides are strongly suppressed ( Fig. 1e ), indicating a dramatic softening of effective magnetic exchange coupling (inset Fig. 1h ). Therefore, high- T c superconductivity is likely associated with two ingredients: a large effective magnetic exchange coupling [15] , much like the large Debye energy for high- T c BCS superconductors, and a strong itinerant electrons-spin excitations coupling from the Fermi surface nesting [10] , similar to electron-phonon coupling in BCS superconductors. Electron and hole-doping evolution of spin excitations To substantiate the key conclusions of Fig. 1 , we present the two-dimensional (2D) constant-energy images of spin excitations in the ( H , K ) plane at different energies for KFe 2 As 2 ( Fig. 3a–c ), Ba 0.67 K 0.33 Fe 2 As 2 ( Fig. 3d–f ), and BaFe 1.7 Ni 0.3 As 2 ( Fig. 3g–i ) above T c . In previous INS work on KFe 2 As 2 , longitudinal incommensurate spin excitations were found by triple axis spectrometer measurements for energies from 3 to 14 meV in the normal state [19] . While we confirmed the earlier work using time-of-flight INS for energies below E =15±1 meV ( Fig. 3a,b ), our new data collected at higher excitation energies reveal that incommensurate spin excitations converge into a broad spin excitation near E =20 meV and disappear for energies above 25 meV ( Fig. 3c ; Supplementary Fig. S1 ). For Ba 0.67 K 0.33 Fe 2 As 2 , spin excitations at E =5±1 meV are longitudinally elongated from Q AF as expected from the DFT calculations ( Fig. 3d ) [18] , [23] . At the resonance energy ( E =15±1 meV) [16] , spin excitations are isotropic above T c ( Fig. 3e ). On increasing energy further to E =50±10 meV, spin excitations change to transversely elongated from Q AF similar to spin excitations in optimally electron-doped superconductor BaFe 1.9 Ni 0.1 As ( Fig. 3f ) [24] . 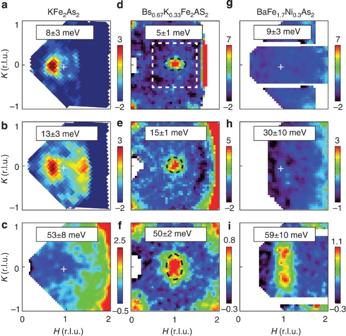Figure 3: Constant-energy slices through magnetic excitations of iron pnictides at different energies. The colour bars represent the vanadium normalized absolute spin excitation intensity in the units of mbarn sr−1meV−1f.u.−1. 2D images of spin excitations at 5 K for KFe2As2(a)E=8±3 meV obtained withEi=20 meV. The right side incommensurate peak is obscured by background scattering. (b) 13±3 meV withEi=35 meV, (c) 53±10 meV withEi=80 meV. For Ba0.67K0.33Fe2As2atT=45 K, images of spin excitations at (d)E=5±1 meV obtained withEi=20 meV, (e) 15±1 meV withEi=35 meV, and (f) 50±2 meV obtained withEi=80 meV. The dashed box in (d) indicates the AF zone boundaries for a single FeAs layer and the black dashed lines mark the orientations of spin excitations at different energies. Images of spin excitations for BaFe1.7Ni0.3As2atT=5 K and (g)E=9±3 meV obtained withEi=80 meV, (h) 30±10 meV withEi=450 meV, and (i) 59±10 meV withEi=250 meV. The white crosses indicate the position ofQAF. Figure 3g–i summarizes similar 2D constant-energy images of spin excitations for nonsuperconducting BaFe 1.7 Ni 0.3 As. At E =9±3 ( Fig. 3g ) and 30±10 meV ( Fig. 3h ), there are no correlated spin excitations near the Q AF . Upon increasing energy to E =59±10 meV ( Fig. 3i ), we see clear spin excitations transversely elongated from Q AF ( Fig. 3i ; Supplementary Fig. S2 ). To further illustrate the presence of a large spin gap in BaFe 1.7 Ni 0.3 As, we compare spin waves in BaFe 2 As 2 [13] and paramagnetic spin excitations in BaFe 1.7 Ni 0.3 As. 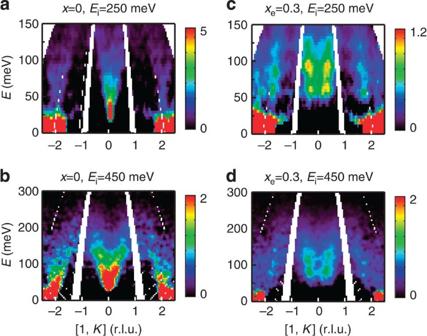Figure 4: The dispersion of spin excitations for BaFe2−xNixAs2along the [1,K] direction. (a,b) The dispersion cuts of BaFe2As2withEi=250 meV andEi=450 meV along [1,K] direction. The data are from MAPS13. (c,d) Identical dispersion cuts of BaFe1.7Ni0.3As2(xe=0.3) at MAPS. Figure 4a,b shows the background subtracted spin wave scattering of BaFe 2 As 2 for the E i =250, 450 meV data, respectively, projected in the wave vector ( Q =[1, K ]) and energy space at 7 K [13] . Sharp spin waves are seen to stem from the AF ordering wave vector Q AF =(1,0) above the ~15 meV spin gap [45] . Figure 4c,d shows identical projections for spin excitations of BaFe 1.7 Ni 0.3 As at 5 K. A large spin gap of ~50 meV is clearly seen in the data near Q AF =(1,0). A detailed comparison of spin excitations in BaFe 2− x Ni x As 2 with x e =0, 0.1, 0.3 is made in Supplementary Figs S3 and S4 . Figure 3: Constant-energy slices through magnetic excitations of iron pnictides at different energies. The colour bars represent the vanadium normalized absolute spin excitation intensity in the units of mbarn sr −1 meV −1 f.u. −1 . 2D images of spin excitations at 5 K for KFe 2 As 2 ( a ) E =8±3 meV obtained with E i =20 meV. The right side incommensurate peak is obscured by background scattering. ( b ) 13±3 meV with E i =35 meV, ( c ) 53±10 meV with E i =80 meV. For Ba 0.67 K 0.33 Fe 2 As 2 at T =45 K, images of spin excitations at ( d ) E =5±1 meV obtained with E i =20 meV, ( e ) 15±1 meV with E i =35 meV, and ( f ) 50±2 meV obtained with E i =80 meV. The dashed box in ( d ) indicates the AF zone boundaries for a single FeAs layer and the black dashed lines mark the orientations of spin excitations at different energies. Images of spin excitations for BaFe 1.7 Ni 0.3 As 2 at T =5 K and ( g ) E =9±3 meV obtained with E i =80 meV, ( h ) 30±10 meV with E i =450 meV, and ( i ) 59±10 meV with E i =250 meV. The white crosses indicate the position of Q AF . Full size image Figure 4: The dispersion of spin excitations for BaFe 2− x Ni x As 2 along the [1, K ] direction. ( a , b ) The dispersion cuts of BaFe 2 As 2 with E i =250 meV and E i =450 meV along [1, K ] direction. The data are from MAPS [13] . ( c , d ) Identical dispersion cuts of BaFe 1.7 Ni 0.3 As 2 ( x e =0.3) at MAPS. 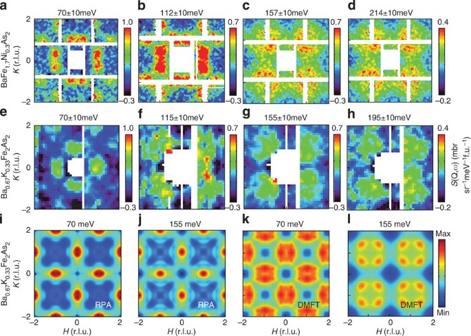Figure 5: Constant-energy images of spin excitations of iron pnictides and its comparison with RPA/DMFT calculations. Spin excitations of BaFe1.7Ni0.3As2in the 2D [H,K] plane at energy transfers of (a)E=70±10 meV obtained withEi=250 meV; (b) 112±10 meVEi=250 meV; (c) 157±10 meV and (d) 214±10 meV withEi=450 meV. All obtained at 5 K. A flat backgrounds have been subtracted from the images. Spin excitations of Ba0.67K0.33Fe2As2at energy transfers of (e)E=70±10 meV obtained withEi=170 meV; (f) 115±10 meV; (g) 155±10 meV; (h) 195±10 meV obtained withEi=450 meV, all at 9 K. Wave vector dependent backgrounds have been subtracted from the images. RPA calculations25of spin excitations for Ba0.67K0.33Fe2As2at (i)E=70 meV and (j)E=155 meV. DMFT calculations24,42for Ba0.67K0.33Fe2As2at (k)E=70 meV and (l)E=155 meV. Full size image Figure 5a–d shows 2D images of spin excitations in BaFe 1.7 Ni 0.3 As 2 at E =70±10, 112±10, 157±10, and 214±10 meV, respectively. Figure 5e–h shows wave vector dependence of spin excitations at energies E =70±10, 115±10, 155±10 and 195±10 meV, respectively, for Ba 0.67 K 0.33 Fe 2 As 2 . Similar to spin waves in BaFe 2 As 2 (ref. 13 ), spin excitations in BaFe 1.7 Ni 0.3 As 2 and Ba 0.67 K 0.33 Fe 2 As 2 split along the K -direction for energies above 80 meV and form rings around Q =(±1,±1) positions near the zone boundary, albeit at slightly different energies. Comparing spin excitations in Fig. 5a–d for BaFe 1.7 Ni 0.3 As 2 with those in Fig. 5e–h for Ba 0.67 K 0.33 Fe 2 As 2 in absolute units, we see that spin excitations in BaFe 1.7 Ni 0.3 As 2 extend to slightly higher energies and have larger intensity above 100 meV. Figure 5: Constant-energy images of spin excitations of iron pnictides and its comparison with RPA/DMFT calculations. Spin excitations of BaFe 1.7 Ni 0.3 As 2 in the 2D [ H,K ] plane at energy transfers of ( a ) E =70±10 meV obtained with E i =250 meV; ( b ) 112±10 meV E i =250 meV; ( c ) 157±10 meV and ( d ) 214±10 meV with E i =450 meV. All obtained at 5 K. A flat backgrounds have been subtracted from the images. Spin excitations of Ba 0.67 K 0.33 Fe 2 As 2 at energy transfers of ( e ) E =70±10 meV obtained with E i =170 meV; ( f ) 115±10 meV; ( g ) 155±10 meV; ( h ) 195±10 meV obtained with E i =450 meV, all at 9 K. Wave vector dependent backgrounds have been subtracted from the images. RPA calculations [25] of spin excitations for Ba 0.67 K 0.33 Fe 2 As 2 at ( i ) E =70 meV and ( j ) E =155 meV. DMFT calculations [24] , [42] for Ba 0.67 K 0.33 Fe 2 As 2 at ( k ) E =70 meV and ( l ) E =155 meV. Full size image As discussed in the spin wave measurements of BaFe 2 As 2 (ref. 13 ), the magnon band top energy at Q =(1,1) governs the effective magnetic exchange couplings J ( J 1a , J 1b , and J 2 ). To estimate the change of J for hole-doped Ba 0.67 K 0.33 Fe 2 As 2 , we calculate the energy cut at Q =(1,1) by exploring the Heisenberg Hamiltonian of the parent compound. It turns out that J 1a , J 1b , and J 2 have comparable effect on the band top. On the basis of the dispersion of Ba 0.67 K 0.33 Fe 2 As 2 , the effective magnetic exchange J is found to be about 10% smaller for Ba 0.67 K 0.33 Fe 2 As 2 compared with that of BaFe 2 As 2 ( Fig. 6 ). For comparison, if we assume the band top for KFe 2 As 2 is around E =25 meV, the effective magnetic exchange should be about 90% smaller for KFe 2 As 2 . Of course, we know this is not an accurate estimation since spin excitations in KFe 2 As 2 are incommensurate and have an inverse dispersion. In any case, given the zone boundary energy of E ≈25 meV ( Supplementary Fig. S1 ), the effective magnetic exchange couplings in KFe 2 As 2 must be much smaller than that of BaFe 2 As 2 . 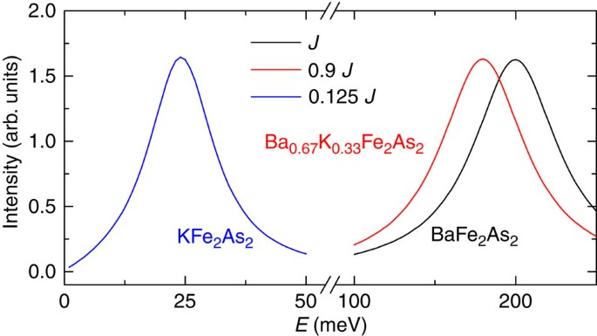Figure 6: The effect of magnetic exchange couplingsJ(J1a,J1bandJ2) on the band top of spin excitations. The black line is energy cut at (0.8<H<1.2, 0.8<K<1.2) r.l.u for BaFe2As2in the Heisenberg spin wave model13. The red line is for Ba0.67K0.33Fe2As2with 10 % soften band top. The blue line is a similar estimation for KFe2As2assuming zone boundary is aroundE=25 meV. Figure 6: The effect of magnetic exchange couplings J ( J 1a , J 1b and J 2 ) on the band top of spin excitations. The black line is energy cut at (0.8< H <1.2, 0.8< K <1.2) r.l.u for BaFe 2 As 2 in the Heisenberg spin wave model [13] . The red line is for Ba 0.67 K 0.33 Fe 2 As 2 with 10 % soften band top. The blue line is a similar estimation for KFe 2 As 2 assuming zone boundary is around E =25 meV. Full size image Theoretical calculations of spin excitations To understand the wave vector dependence of spin excitations in hole-doped Ba 0.67 K 0.33 Fe 2 As 2 , we have carried out the random phase approximation (RPA) calculation of the dynamic susceptibility in a pure itinerant electron picture using the method described before [25] . Figure 5i,j shows RPA calculations of spin excitations at E =70 and 155 meV, respectively, for Ba 0.67 K 0.33 Fe 2 As 2 assuming that hole doping induces a rigid band shift [25] . While a pure RPA type itinerant model can explain longitudinally elongated spin excitations at low-energies [18] , it clearly fails to describe the transversely elongated spin excitations in hole-doped iron pinctides at high energies ( Fig. 5e,g ). For comparison with the RPA calculation, we also used a combined DFT and DMFT approach [24] , [42] to calculate the imaginary part of the dynamic susceptibility χ ″ ( Q ,ω) in the paramagnetic state. Figure 5k,i shows calculated spin excitations at E =70 and 155 meV, respectively. Although the model still does not agree in detail with the data in Fig. 5e,g , it captures the trend of spectral weight transfer away from Q AF =(1,0) on increasing energy and forming a pocket centred at Q =(1,1). Dispersions of spin excitations and local dynamic susceptibility By carrying out cuts through the 2D images similar to Figs 3d–f and 5e–h along the [1, K ] and [ H ,0] directions ( Supplementary Figs S5 and S6 ), we establish the spin excitation dispersion along the two high symmetry directions for Ba 0.67 K 0.33 Fe 2 As 2 and compare with the dispersion of BaFe 2 As 2 ( Fig. 1f ) [13] . In contrast to the dispersion of electron-doped BaFe 1.9 Ni 0.1 As 2 (ref. 24 ), we find clear softening of the zone boundary spin excitations in hole-doped Ba 0.67 K 0.33 Fe 2 As 2 from spin waves in BaFe 2 As 2 (ref. 13 ). We estimate that the effective magnetic exchange coupling in Ba 0.67 K 0.33 Fe 2 As 2 is reduced by about 10% from that of BaFe 2 As 2 ( Fig. 6 ). Similarly, Fig. 1g shows the dispersion curve of BaFe 1.7 Ni 0.3 As 2 along the [1, K ] direction plotted together with that of BaFe 2 As 2 (ref. 13 ). For energies below ~50 meV, spin excitations are completely gapped marked in the dashed area probably due to the missing hole-electron Fermi pocket quasiparticle excitations [40] . On the basis of the 2D spin excitation images similar to Fig. 3a–c ; we plot in Fig. 1e the dispersion of incommensurate spin excitations in KFe 2 As 2 . The incommensurability of spin excitations is weakly energy dependent below E =12 meV but becomes smaller with increasing energy above 12 meV. Correlated spin excitations for energies above 25 meV are suppressed as shown in the shaded area in Fig. 1e . To quantitatively determine the effect of electron and hole doping on the overall spin excitations spectra, we calculate the local dynamic susceptibility per formula unit (f.u.) in absolute units, defined as χ ″ ( ω )=∫χ ″ ( q ,ω) d q /∫ d q (ref. 24 ), where , at different energies for Ba 0.67 K 0.33 Fe 2 As 2 , BaFe 1.7 Ni 0.3 As 2 , and KFe 2 As 2 . Figure 1h shows the outcome together with previous data on optimally electron-doped superconductor BaFe 1.9 Ni 0.1 As 2 (ref. 24 ). While electron doping up to BaFe 1.7 Ni 0.3 As 2 does not change much the spectral weight of high-energy spin excitations from that of BaFe 1.9 Ni 0.1 As 2 , hole-doping dramatically suppresses the high-energy spin excitations and shift the spectral weight to lower energies ( Fig. 1h ). For heavily hole-doped KFe 2 As 2 , spin excitations are mostly confined to energies below about E =25 meV (inset in Fig. 1h ). The solid green, red, black, and blue lines in Fig. 7 show calculated local susceptibility in absolute units based on a combined DFT and DMFT approach for KFe 2 As 2 , Ba 0.67 K 0.33 Fe 2 As 2 , BaFe 2 As 2 , and BaFe 1.9 Ni 0.1 As 2 [24] , respectively. This theoretical method predicts that electron doping to BaFe 2 As 2 does not affect the spin susceptibility at high energy ( E >150 meV), while spin excitations in the hole-doped compound beyond 100 meV are suppressed by shifting the spectral weight to lower energies. This is in qualitative agreement with our absolute intensity measurements ( Fig. 1h ). The reduction of the high-energy spin spectral weight and its transfer to low energy with hole doping, but not with electron doping, is not naturally explained by the band theory ( Fig. 7 ) and requires models that incorporate both the itinerant quasiparticles and the local moment physics [9] , [42] . The hole doping makes the electronic state more correlated, as local moment formation is strongest in the half-filled d 5 shell, and mass enhancement larger thereby reducing the electronic energy scale in the problem. The dashed lines in Fig. 7 show the results of calculated local susceptibility using RPA, which clearly fails to describe the electron- and hole-doping dependence of the local susceptibility. 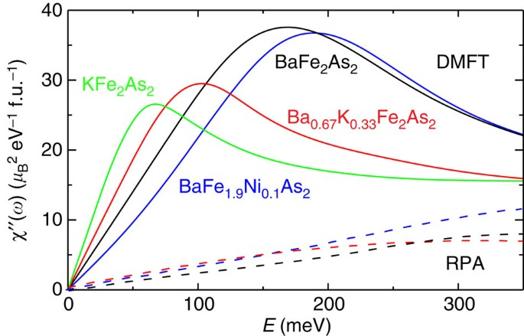Figure 7: RPA and LDA+DMFT calculated local susceptibility for different iron pnictides. RPA and LDA+DMFT calculations of χ″(ω) in absolute units for KFe2As2and Ba0.67K0.33Fe2As2comparing with earlier results for BaFe2As2and BaFe1.9Ni0.1As224. Figure 7: RPA and LDA+DMFT calculated local susceptibility for different iron pnictides. RPA and LDA+DMFT calculations of χ ″ (ω) in absolute units for KFe 2 As 2 and Ba 0.67 K 0.33 Fe 2 As 2 comparing with earlier results for BaFe 2 As 2 and BaFe 1.9 Ni 0.1 As 2 [24] . Full size image Estimation of the superconductivity-induced magnetic exchange energy Finally, to determine how low-energy spin excitations are coupled to superconductivity in Ba 0.67 K 0.33 Fe 2 As 2 , we carried out a detailed temperature-dependent study of spin excitation at E =15±1 meV. Comparing with strongly c axis modulated low-energy ( E <7 meV) spin excitations [18] , spin excitations at the resonance energy are essentially 2D without much c axis modulations. In previous work [18] , we have shown that spin excitations near the neutron spin resonance are longitudinally elongated and change dramatically in intensity across T c . However, these measurements are obtained in arbitrary units and therefore cannot be used to determine the magnetic exchange energy. 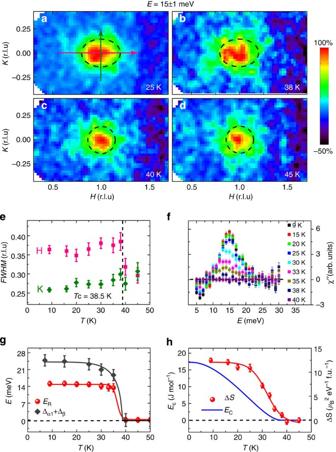Figure 8: Properties of the resonance acrossTc=38.5 K for Ba0.67K0.33Fe2As2. Constant-energy (E=15±1 meV) images of spin excitations at (a)T=25, (b) 38, (c) 40, and (d) 45 K obtained withEi=35 meV. In order to make fair comparison of the scattering line shape at different temperatures, the peak intensity at each temperature is normalized to 1. The pink and green arrows in (a) mark wave vector cut directions across the resonance. The integration ranges are −0.2≤K≤0.2 along the [H,0] direction and 0.8≤H≤1.2 along the [1,K] direction. The full-width-at-half-maximum (FWHM) of spin excitations are marked as dashed lines. (e) The FWHM of the resonance along the [H,0] and [1,K] directions as a function of temperature acrossTc. (f) Energy dependence of the resonance obtained by subtracting the low-temperature data from the 45 K data, and correcting for the Bose population factor. (g) The black diamonds show temperature dependence of the sum of hole and electron pocket electronic gaps obtained from Angle Resolved Photoemission experiments for Ba0.67K0.33Fe2As2(ref.40). The red solid circles show temperature dependence of the resonance. (h) Temperature dependence of the superconducting condensation energy from heat capacity measurements43and the intensity of the resonance integrated from 14–16 meV. The error bars indicate the statistical errors of one s.d. Figure 8a–d shows the 2D mapping of the resonance at T =25, 38, 40, and 45 K, respectively. While the resonance reveals a clear oval shape at temperatures below T c consistent with earlier work ( Fig. 8a,b ) [18] , it changes into an isotropic circular shape abruptly at T c ( Fig. 8c,d ) as shown by the dashed lines representing full-width-at-half-maximum of the excitations ( Supplementary Fig. S7 ). Temperature dependence of the resonance width along the [ H ,0] and [1, K ] directions in Fig. 8e reveals that the isotropic to anisotropic transition in momentum space occurs at T c . Figure 8f shows temperature dependence of the resonance from 9–40 K, which vanishes at T c . Figure 8g plots temperature dependence of the mode energy together with the sum of the superconducting gaps from the hole and electron pockets [40] . Figure 8h compares temperature dependence of the superconducting condensation energy [43] with superconductivity-induced intensity gain of the resonance. By calculating spin excitations induced changes in magnetic exchange energy using equation (1) (see Methods and Supplementary Fig. S8 ) [15] , we find that the difference of magnetic exchange interaction energy between the superconducting and normal state is approximately seven times larger than the superconducting condensation energy [43] , thus indicating that AF spin excitations can be the major driving force for superconductivity in Ba 0.67 K 0.33 Fe 2 As 2 . Figure 8: Properties of the resonance across T c =38.5 K for Ba 0.67 K 0.33 Fe 2 As 2 . Constant-energy ( E =15±1 meV) images of spin excitations at ( a ) T =25, ( b ) 38, ( c ) 40, and ( d ) 45 K obtained with E i =35 meV. In order to make fair comparison of the scattering line shape at different temperatures, the peak intensity at each temperature is normalized to 1. The pink and green arrows in ( a ) mark wave vector cut directions across the resonance. The integration ranges are −0.2≤ K ≤0.2 along the [ H ,0] direction and 0.8≤ H ≤1.2 along the [1, K ] direction. The full-width-at-half-maximum (FWHM) of spin excitations are marked as dashed lines. ( e ) The FWHM of the resonance along the [ H ,0] and [1, K ] directions as a function of temperature across T c . ( f ) Energy dependence of the resonance obtained by subtracting the low-temperature data from the 45 K data, and correcting for the Bose population factor. ( g ) The black diamonds show temperature dependence of the sum of hole and electron pocket electronic gaps obtained from Angle Resolved Photoemission experiments for Ba 0.67 K 0.33 Fe 2 As 2 (ref. 40 ). The red solid circles show temperature dependence of the resonance. ( h ) Temperature dependence of the superconducting condensation energy from heat capacity measurements [43] and the intensity of the resonance integrated from 14–16 meV. The error bars indicate the statistical errors of one s.d. Full size image One way to quantitatively estimate the impact of hole/electron doping and superconductivity to spin waves of BaFe 2 As 2 is to determine the energy dependence of the local moment and total fluctuating moments ‹ m 2 › (ref. 24 ). From Fig. 1h , we see that hole-doping suppresses high-energy spin waves of BaFe 2 As 2 and pushes the spectral weight to resonance at lower energies. The total fluctuating moment of Ba 0.67 K 0.33 Fe 2 As 2 below 300 meV is ‹ m 2 ›=1.7±0.3 per Fe, somewhat smaller than per Fe for BaFe 2 As 2 and BaFe 1.9 Ni 0.1 As 2 (ref. 24 ). For comparison, BaFe 1.7 Ni 0.3 As 2 and KFe 2 As 2 have ‹ m 2 ›=2.74±0.11 and per Fe, respectively. Therefore, the total magnetic spectral weights for different iron pnictides have no direct correlation with their superconducting T c s. Table 1 summarizes the comparison of effective magnetic exchange couplings, total fluctuating moments, and spin excitation band widths for BaFe 2− x Ni x As 2 with x e =0,0.1,0.3 and Ba 1− x K x Fe 2 As 2 with x h =0.33, 1. Table 1 Summary of properties of various iron pnictides. Full size table From Fig. 1h , we also see that the spectral weight of the resonance and low-energy (<100 meV) magnetic scattering in Ba 0.67 K 0.33 Fe 2 As 2 is much larger than that of electron-doped BaFe 1.9 Ni 0.1 As 2 . This is consistent with a large superconducting condensation energy in Ba 0.67 K 0.33 Fe 2 As 2 since its effective magnetic exchange coupling J is only ~10% smaller than that of BaFe 1.9 Ni 0.1 As 2 ( Fig. 1h ) [43] , [46] . For electron-overdoped nonsuperconducting BaFe 1.7 Ni 0.3 As 2 , the lack of superconductivity is correlated with the absence of low-energy spin excitations coupled to the hole and electron Fermi surface nesting even though the effective magnetic exchange couplings remain large [40] , [41] . This means that by eliminating [‹ S i + x · S i › N −‹ S i + x · S i › S ], there is no magnetic driven superconducting condensation energy, and thus no superconductivity. On the other hand, although the suppression of correlated high-energy spin excitations in KFe 2 As 2 can dramatically reduce the effective magnetic exchange coupling in KFe 2 As 2 ( Figs 1e and 6 ), one can still have superconductivity with reduced T c . If spin excitations are a common thread of the electron pairing interactions for unconventional superconductors [15] , our results reveal that the large effective magnetic exchange couplings and itinerant electron-spin excitation interactions may both be important ingredients to achieve high- T c superconductivity, much like the large Debye energy and the strength of electron-lattice coupling are necessary for high- T c BCS superconductors. Therefore, our data indicate a possible correlation between the overall magnetic excitation band width, the presence of low-energy spin excitations, and the scale of T c . This suggests that both high-energy spin excitations and low-energy spin excitation itinerant electron coupling are important for high- T c superconductivity. Sample preparation Single crystals of Ba 0.67 K 0.33 Fe 2 As 2 , KFe 2 As 2 , and BaFe 1.7 Ni 0.3 As 2 are grown using the flux method [18] , [25] . The actual crystal compositions were determined using the inductively coupled plasma analysis. We coaligned 19 g of single crystals of Ba 0.67 K 0.33 Fe 2 As 2 (with in-plane and out-of-plane mosaic of 4°), 3 g of KFe 2 As 2 (with in-plane and out-of-plane mosaic of ~7.5°), and 40 g of BaFe 1.7 Ni 0.3 As 2 (with in-plane and out-of-plane mosaic of ~3°). Neutron scattering experiments Our INS experiments were carried out on the MERLIN and MAPS time-of-flight chopper spectrometers at the Rutherford-Appleton Laboratory, UK [13] , [24] . Various incident beam energies were used as specified, and mostly with E i parallel to the c axis. To facilitate easy comparison with spin waves in BaFe 2 As 2 (ref. 13 ), we defined the wave vector Q at ( q x , q y , q z ) as ( H , K , L )=( q x a o /2π, q y b o /2π, q z c /2π) reciprocal lattice units (rlu) using the orthorhombic unit cell, where a o ≈ b o =5.57 Å, and c =13.135 Å for Ba 0.67 K 0.33 Fe 2 As 2 , a o ≈ b o =5.43 Å, and c =13.8 Å for KFe 2 As 2 , and a o = b o =5.6 Å, and c =12.96 Å for BaFe 1.7 Ni 0.3 As 2 . The data are normalized to absolute units using a vanadium standard with 20% errors [24] and confirmed by acoustic phonon normalization (see Supplementary Note 1 ). Supplementary Discussion provides additional data analysis on electron-doped iron pnictides, focusing on the comparison of electron overdoped nonsuperconducting BaFe 1.3 Ni 0.3 As 2 with optimally electron-doped superconductor BaFe 1.9 Ni 0.1 As 2 and AF BaFe 2 As 2 . DFT+DMFT calculations Our theoretical DFT+DMFT method for computing the magnetic excitation spectrum employs the ab initio full potential implementation of the method, as detailed in ref. 47 . The DFT part is based on the code of Wien2k [48] . The DMFT method requires solution of the generalized quantum impurity problem, which is here solved by the numerically exact continuous-time quantum Monte Carlo method [49] , [50] . The Coulomb interaction matrix for electrons on iron atom was determined by the self-consistent GW method in Kutepov et al. [51] , giving U =5 eV and J =0.8 eV for the local basis functions within the all electron approach employed in our DFT+DMFT method. The dynamical magnetic susceptibility χ ″ ( Q , E ) is computed from the ab initio perspective by solving the Bethe-Salpeter equation, which involves the fully interacting one particle Greens function computed by DFT+DMFT, and the two-particle vertex, also computed within the same method (for details see Park et al. [42] ). We computed the two-particle irreducible vertex functions of the DMFT impurity model, which coincides with the local two-particle irreducible vertex within the DFT+DMFT method. The latter is assumed to be local in the same basis in which the DMFT self-energy is local, here implemented by projection to the muffin-tin sphere. Calculation of magnetic exchange energy and superconducting condensation energy for Ba 0.67 K 0.33 Fe 2 As 2 In a neutron scattering experiment, we measure scattering function S ( Q , E = ħ ω) which is related to the imaginary part of the dynamic susceptibility via S ( Q ,ω)=[1+ n (ω, T )]χ ″ ( Q ,ω), where n (ω, T ) is the Bose population factor. The magnetic exchange coupling and the imaginary part of spin susceptibility are related via the formula [15] : where g =2 is the Landé g -factor. Hence, we are able to obtain the change in magnetic exchange energy between the superconducting and normal states by the experimental data of χ ″ ( Q ,ω) in both states using equation (1). Strictly speaking, we want to estimate the zero temperature difference of the magnetic exchange energy between the normal and the superconducting states, and use the outcome to compare with the superconducting condensation energy [15] . Unfortunately, we do not have direct information on the normal state χ ″ ( Q ,ω) at zero temperature. Nevertheless, since our neutron scattering measurements at low-energies showed that the χ ″ ( Q ,ω) are very similar below and above T c near the AF wave vector Q AF =(1,0,1) and only a very shallow spin gap at Q =(1,0,0) (see Fig. 1f,h in Zhang et al. [18] ), we assume that there are negligible changes in χ ″ ( Q ,ω) above and below T c at zero temperature for energies below 5 meV. For spin excitation energies above 6 meV, the Bose population factors between 7 and 45 K are negligibly small. In previous work on optimally doped YBa 2 Cu 3 O 6.95 superconductor, we have assumed that spin excitations in the normal state at zero temperature are negligibly small and thus do not contribute to the exchange energy [30] . The directly measured quantity is the scattering differential cross section where k i and k f are the magnitudes of initial and final neutron momentum and F ( Q ) is the Fe 2+ magnetic form factor, and (γ r e ) 2 =0.2905, barn·sr −1 . The quantity χ ″ ( Q , E ) in both superconducting and normal states can be fitted by a Gaussian for resonance wave vector (1,0) and by cutting the raw data. The outcome is summarized in the Supplementary Table S1 , where the unit of E is meV and that of A s(n) is mbarn˙meV −1 ·sr −1 ·Fe −1 . For the case below 5 meV, we assume that A n decreases to zero linearly with energy and A s = A n (see Fig. 1h in Zhang et al. [18] ), while the σ keeps the value at 5 meV. The assumption is shown in Supplementary Figure S8 , where the resonance is seen at E =15 meV. Because the condensation energy is only defined at zero temperature, we take T =0 in the formula equation (3) and the integral gives: The magnetic exchange coupling constants in an anisotropic model are estimated to be which are 10% smaller than that of BaFe 2 As 2 (ref. 13 ) and we estimate S to be close to ½ (ref. 24 ). Hence the exchange energy change is The condensation energy U c for optimally doped Ba 0.67 K 0.33 Fe 2 As 2 can be calculated to be from the specific heat data of Popovich et al. [43] Therefore, we have the ratio Δ E ex / U c ≈7.4, meaning that the change in the magnetic exchange energy is sufficient to account for the superconducting condensation energy in Ba 0.67 K 0.33 Fe 2 As 2 . How to cite this article: Wang, M. et al. Doping dependence of spin excitations and its correlations with high-temperature superconductivity in iron pnictides. Nat. Commun. 4:2874 doi: 10.1038/ncomms3874 (2013).